Natural variation in timing of stress-responsive gene expression predicts heterosis in intraspecific hybrids ofArabidopsis The genetic distance between hybridizing parents affects heterosis; however, the mechanisms for this remain unclear. Here we report that this genetic distance correlates with natural variation and epigenetic regulation of circadian clock-mediated stress responses. In intraspecific hybrids of Arabidopsis thaliana , genome-wide expression of many biotic and abiotic stress-responsive genes is diurnally repressed and this correlates with biomass heterosis and biomass quantitative trait loci. Expression differences of selected stress-responsive genes among diverse ecotypes are predictive of heterosis in their hybrids. Stress-responsive genes are repressed in the hybrids under normal conditions but are induced to mid-parent or higher levels under stress at certain times of the day, potentially balancing the tradeoff between stress responses and growth. Consistent with this hypothesis, repression of two candidate stress-responsive genes increases growth vigour. Our findings may therefore provide new criteria for effectively selecting parents to produce high- or low-yield hybrids. Hybrid plants and animals, such as corn and domestic dogs, grow larger and more vigourously than their parents, a common phenomenon known as hybrid vigour or heterosis. Since Darwin [1] systematically described the phenomenon, heterosis has been widely applied in agriculture to dramatically improve the production of crops and farm animals [2] , [3] . However, the molecular basis for heterosis remains elusive [4] , [5] , and traditional dominance and overdominance genetic models cannot adequately explain heterosis in yeast and many crop plants [3] , [5] , [6] , [7] , [8] . Heterosis in food crops often refers to grain yield, while biomass heterosis is commonly measured in other crops including vegetable and energy crops. In this study, heterosis and biomass heterosis are used interchangeably. A common observation is the positive correlation between genetic divergence levels in parents and levels of heterosis in hybrids [3] , [5] , [8] , [9] , [10] . This suggests an underlying mechanism that allows hybrids to utilize the genetic divergence between the parents to promote heterosis [10] , [11] . This genetic divergence is probably reflected in the natural variation of gene expression between parents, which results from generations of selection and/or adaptation to local environments with variable diurnal and stress conditions [12] , [13] . Indeed, matching gene expression rhythms with light–dark cycles promotes growth and fitness in plants and animals [14] , [15] , [16] and heterosis in Arabidopsis allopolyploids and hybrids [17] . In Arabidopsis thaliana , the RNA-directed DNA methylation pathway mediates a parent-of-origin effect on circadian rhythms, leading to biomass heterosis in reciprocal F1 hybrids [18] . In A. thaliana diploids, the circadian clock regulates abiotic [19] , [20] and biotic [21] , [22] , [23] stress responses. However, there is a tradeoff between stress responses and fitness; constitutive expression of stress-responsive genes reduces fitness and growth [24] , [25] , while repressing disease resistance genes promotes growth [26] . In Arabidopsis allotetraploids derived from interspecific hybrids between A. thaliana and A. arenosa , the increased growth vigour is associated with the repression of many stress-responsive genes [27] , consistent with the tradeoff between growth and stress response in the diploids [24] , [25] , [28] . Here we performed genome-wide gene expression analysis and investigated mechanistic insights into natural variation and timing of stress-responsive gene expression in heterosis. We found that stress-responsive gene expression levels between parents could serve as a genetic indicator to predict biomass heterosis in hybrids, supporting the aforementioned concept. Diurnal repression of stress-responsive genes in hybrids To assess the role of diurnal stress-responsive gene expression in heterosis, we deep-sequenced mRNAs from 3-week-old seedling leaves of highly heterotic F1 hybrids between A. thaliana Col and C24 ecotypes at zeitgeber time (ZT) 0 (dawn), ZT6 (midday) and ZT15 (dusk) [29] , [30] ( Fig. 1a ). All experiments were performed under diurnal conditions where heterosis naturally occurs. 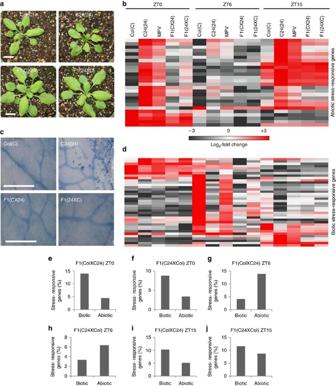Figure 1: Expression of stress-responsive genes is altered in reciprocal F1 hybrids. Expression in hybrids is compared with parents (by convention, the female is listed first in a genetic cross). (a,c) Rosettes of 3-week-old plants (scale bars, 1 cm) (a) and the tenth leaf stained with Trypan blue (scale bars, 0.5 mm;c). (b,d) Clustered heatmaps of RNA-seq data (Supplementary Data 2) showing subsets of genes in biotic (b) and abiotic (d) stress (ZT0=dawn). Fold-change: log2-transformed values from low (dark grey) to high (red). (e–j) Percentage of downregulated differentially expressed genes that are biotic or abiotic stress-responsive genes at ZT0 (e,f), ZT6 (g,h) and ZT15 (i,j) in reciprocal F1 hybrids ColXC24 (e,g,i) and C24XCol (f,h,j). Figure 1: Expression of stress-responsive genes is altered in reciprocal F1 hybrids. Expression in hybrids is compared with parents (by convention, the female is listed first in a genetic cross). ( a , c ) Rosettes of 3-week-old plants (scale bars, 1 cm) ( a ) and the tenth leaf stained with Trypan blue (scale bars, 0.5 mm; c ). ( b , d ) Clustered heatmaps of RNA-seq data ( Supplementary Data 2 ) showing subsets of genes in biotic ( b ) and abiotic ( d ) stress (ZT0=dawn). Fold-change: log 2 -transformed values from low (dark grey) to high (red). ( e – j ) Percentage of downregulated differentially expressed genes that are biotic or abiotic stress-responsive genes at ZT0 ( e , f ), ZT6 ( g , h ) and ZT15 ( i , j ) in reciprocal F1 hybrids ColXC24 ( e , g , i ) and C24XCol ( f , h , j ). Full size image The percentage of differentially expressed genes (DEGs) between F1 hybrids and the midparent value (MPV) was highest ( ∼ 5%) at ZT6 (noon), followed by ∼ 3% at ZT0 (dawn), and ∼ 1.3% at ZT15 (dusk; Supplementary Data 1 ). Gene ontology (GO) analysis ( Supplementary Fig. 1a–f ) revealed that both photosynthetic and stress-responsive genes were enriched in the DEGs relative to all expressed genes (DEGseq q -value (false discovery rate (FDR)-adjusted P value) <0.05, see Methods). In all, 30 of 267–328 ( ∼ 10%) genes that were upregulated in reciprocal hybrids at ZT6 belonged to the photosynthetic processes using GO term analysis ( Supplementary Fig. 1g–k ), consistent with previous observations of increased photosynthetic capacity in hybrids [17] , [31] . Note that gene expression patterns were slightly and consistently different between the reciprocal F1 crosses (also below), which is known to be because of parent-of-origin effects on circadian rhythms and biomass heterosis [18] . These differences were not further investigated in this study. Among downregulated genes, 3–13% were in the GO classifications of biotic and abiotic stress-responsive genes ( Fig. 1e–j and Supplementary Data 2 ). The repression of these genes, including 26 known biotic and 38 known abiotic stress-responsive genes (classified using GO term analysis, see Methods), occurred at different times of the day ( Fig. 1b,d ). At ZT6, two- to threefold more abiotic than biotic stress-responsive genes were repressed ( Fig. 1g,h ). This trend was reversed at ZT0 and ZT15, and biotic stress-responsive genes comprised a larger proportion of the repressed genes ( Fig. 1e,f,i,j ). The timing of repression in the hybrids was confirmed using quantitative reverse transcriptase–polymerase chain reaction (qRT–PCR) analysis in two diurnal cycles (48 h) in three biological replicates. Biotic stress-responsive genes such as ACCELERATED CELL DEATH6 ( ACD6 , At4g14400), PATHOGEN AND CIRCADIAN CONTROLLED1 ( PCC1 , At3g22231) and HOMOLOG OF SUGAR BEET HS1 PRO-2 ( HSPRO2 , At2g40000) were primarily repressed to below MPV levels between ZT0 and ZT6 ( Fig. 2a and Supplementary Fig. 2a,b ), and PATHOGENESIS-RELATED GENES1 ( PR1 , At2g14610) and PR5 (At1g75040) were repressed at all times ( Supplementary Fig. 2c,d ). However, cold stress-responsive genes, including COLD-REGULATED78 ( COR78 , At5g52310), COR47 (At1g20440), COR15A (At2g42540), RESPONSIVE-TO-DESICCATION22 ( RD22 , At5g25610) and RD28 (At2g37180), were repressed in the middle and later parts of the day ( Fig. 2b and Supplementary Fig. 2e–h ). A slight shift of the expression peaks between ecotypes may reflect their adaptation to fluctuating local environments. Moreover, expression rhythms of many stress-responsive genes are modulated by other signalling factors in addition to the circadian clock [19] , [21] . 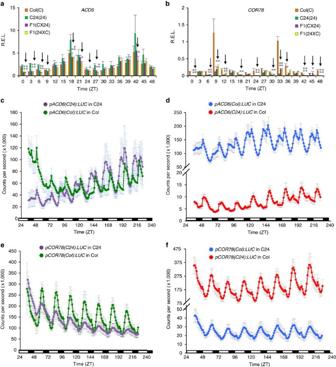Figure 2: Expression of ACD6 and COR78. ACD6andCOR78were subjected to diurnal regulation in two ecotypes, Col and C24, and downregulation in hybrids (arrows). (a,b) Relative expression levels (R.E.L.) ofACD6(a) andCOR78(b) every 3 h in a 48-h period (ZT 0=dawn; mean±s.d., values were averaged from three biological replicates). Single and double asterisks indicate statistical significance levels atP<0.05 andP<0.01 using two-tailed Student’st-test (compared with MPV), respectively. (c,d) Bioluminescent activities (counts per second in 1,000) of transgenic (T2) seedlings that expressedACD6(Col):LUCin Col (green) orACD6(C24):LUCin C24 (purple;c) andACD6(C24):LUCin Col (red) orACD6(Col):LUCin C24 (blue;d). (e,f) Bioluminescent activities of transgenic seedlings that expressedCOR78(Col):LUCin Col (green) orCOR78(C24):LUCin C24 (purple;e) andCOR78(Col):LUCin C24 (blue) orCOR78(C24):LUCin Col (red;f). Diurnal cycles of light (open) and dark (filled) and one of three replicate experiments (mean±s.e.m.,n=16 individuals per transgenic line, three independent transgenic lines were examined) are shown. Figure 2: Expression of ACD6 and COR78. ACD6 and COR78 were subjected to diurnal regulation in two ecotypes, Col and C24, and downregulation in hybrids (arrows). ( a , b ) Relative expression levels (R.E.L.) of ACD6 ( a ) and COR78 ( b ) every 3 h in a 48-h period (ZT 0=dawn; mean±s.d., values were averaged from three biological replicates). Single and double asterisks indicate statistical significance levels at P <0.05 and P <0.01 using two-tailed Student’s t- test (compared with MPV), respectively. ( c , d ) Bioluminescent activities (counts per second in 1,000) of transgenic (T2) seedlings that expressed ACD6(Col):LUC in Col (green) or ACD6(C24):LUC in C24 (purple; c ) and ACD6(C24):LUC in Col (red) or ACD6(Col):LUC in C24 (blue; d ). ( e , f ) Bioluminescent activities of transgenic seedlings that expressed COR78(Col):LUC in Col (green) or COR78(C24):LUC in C24 (purple; e ) and COR78(Col):LUC in C24 (blue) or COR78(C24):LUC in Col (red; f ). Diurnal cycles of light (open) and dark (filled) and one of three replicate experiments (mean±s.e.m., n =16 individuals per transgenic line, three independent transgenic lines were examined) are shown. Full size image This genome-wide repression of stress-responsive genes could be caused by cis - and trans -acting factors in the hybrids, which was tested using all expressed genes [32] , [33] . Consistent with the findings in the interspecific hybrids of Arabidopsis [32] or yeast [33] , >43% more genes exhibited cis- effects than trans -effects in the F1 hybrids at ZT0, ZT6 and ZT15 ( Supplementary Fig. 3a ). However, among stress-responsive genes, significantly more genes displayed trans -effects than cis -effects at all time points (FDR-adjusted P <0.05, hypergeometric test, Supplementary Fig. 3b ). The trans -regulated genes of either parental origin could be repressed to the low-parent level or lower ( Supplementary Fig. 3c–h ), including several known biotic ( Supplementary Fig. 3i–l ) and abiotic ( Supplementary Fig. 3m–p ) stress-responsive genes. The genome-wide data suggest a role for trans -acting factors in the diurnal repression of stress-responsive genes in these hybrids. These trans -acting factors are predicted to involve circadian-clock regulators [10] , as the clock is known to regulate stress-responsive gene expression [19] , [21] . Indeed, DEGs in the hybrids included circadian-regulated genes ( Supplementary Table 1 ), which were significantly enriched with the evening element (EE) ( P =0.018) and CIRCADIAN CLOCK ASSOCIATED1 ( CCA1 , At2g46830)-binding site (CBS) ( P <10 −6 ; Supplementary Data 2 ). The circadian clock regulators, CCA1 and LATE ELONGATED HYPOCOTYL ( LHY , At1g01060), were repressed in the middle of the day and upregulated around dawn ( Supplementary Fig. 4a,b ), and their feedback regulator TOC1 (At5g61380) showed the opposite expression changes ( Supplementary Fig. 4c ), consistent with previous results [17] , [29] . As a result of the clock regulation [20] , [34] , the phases of up- and downregulated DEGs in the hybrids at ZT0 and ZT6 were clustered in the middle of the day and towards dawn, respectively ( Supplementary Fig. 4d–i ). Hence, the expression of many circadian clock-associated genes and stress-responsive genes is coordinately changed, which correlates with growth vigour in the hybrids. Circadian rhythms and stress responses in Arabidopsis Expression level changes in certain stress-responsive genes among different ecotypes may result from plants experiencing different stresses during the day and night, leading to natural variation [19] , [21] , [35] . To determine natural variation of stress-responsive gene expression between ecotypes, we used two well-characterized biotic ( ACD6 ) [26] and abiotic ( COR78 ) [19] stress-responsive genes as examples in stable transgenic plants expressing a promoter:luciferase ( LUC ) reporter. ACD6:LUC and COR78:LUC displayed rhythmic activities in both Col and C24 ecotypes ( Fig. 2c,e ) and showed natural variation in transgene activity between Col and C24, consistent with the expression of endogenous genes ( Fig. 2a,b ). ACD6(C24):LUC in C24 was expressed at higher levels than ACD6(Col):LUC in Col ( Fig. 2c ). Likewise, COR78(Col):LUC in Col was expressed at higher levels than COR78(C24):LUC in C24 ( Fig. 2e ). Notably, the expression differences between the ecotypes were amplified when they were expressed in reciprocal combinations. For instance, ACD6(Col):LUC expression amplitudes in C24 were 10- to 15-fold higher than ACD6(C24):LUC levels in Col ( Fig. 2d ). COR78(C24):LUC amplitudes in Col were seven- to eightfold higher than COR78(Col):LUC in C24 ( Fig. 2f ). Thus, genetic backgrounds could act as trans -acting factors to mediate rhythmic expression peaks of these stress-responsive genes, probably through altered binding of regulatory factors such as the clock proteins or other upstream regulators to the promoters between the ecotypes ( Supplementary Table 2 ). We further tested whether stress conditions affect rhythmic expression and whether the clock regulates expression of stress-responsive genes in the clock mutants as in the wild type [19] , [21] . Since the clock mutants, namely, cca1-1 , lhy21 and cca1-1 1lhy21 , are in the Ws ecotype background, Ws was used as the wild type for comparison with the clock mutants. Salicylic acid (SA), a plant hormone that triggers biotic stress responses [36] , induced elevated arrhythmic expression of ACD6(Ws):LUC in the transgenic plants ( Fig. 3a ). Likewise, cold-shock transiently induced COR78(Ws):LUC expression, but the induction was rhythmic and remained for ∼ 36 h (ref. 37 ; Fig. 3b ). In the absence of stress, the period of ACD6(Ws):LUC activity (24.26±0.30 s.e.m., n =16 individuals per transgenic line) was nearly normal in the cca1-11 or lhy21 mutant, but was shortened by ∼ 1 h in the cca1-1lhy21 double mutant (23.17±0.41, P <0.05, Student's t -test; Fig. 3c ). However, both the expression amplitudes and periods of COR78(Ws):LUC were severely altered in the single ( cca1-11 , 23.73±0.51; lhy21 24.14±0.30, P <0.05) or double (22.61±0.66, P <0.05) mutant ( Fig. 3e ). Under stress conditions, SA-mediated induction of ACD6(Ws):LUC was hindered in the double mutant, but not in the single mutants ( Fig. 3d ). Induction of COR78(Ws):LUC after cold shock was compromised in all mutants tested ( Fig. 3f ). These data indicate that the clock regulators, CCA1 and LHY together, or CCA1 alone, mediate expression amplitudes and periods of these biotic and abiotic stress-responsive genes in stress and non-stress conditions, as previously suggested [21] , [38] , [39] . 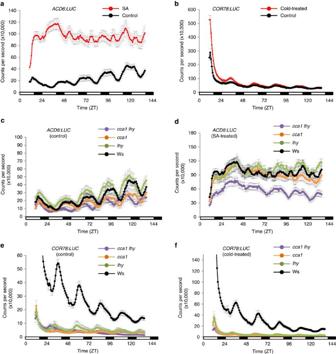Figure 3: The circadian clock regulates the rhythmic expression ofACD6andCOR78. (a,b) Bioluminescent activities ofpACD6(Ws):LUCin T3 transgenic seedlings that were treated with SA (red) and the control (black;a) and ofpCOR78(Ws):LUCin T3 transgenic seedlings that were treated with cold (red) and the control (black;b). (c,d) Altered bioluminescent activities ofpACD6(Ws):LUCin T3 transgenic seedlings incca1-11(orange),lhy21(green),cca1-11 lhy21(purple) and Ws (black) backgrounds, which were sprayed with water (control,c) or SA (d). (e,f) Altered bioluminescent activities ofpCOR78(Ws):LUCin T3 transgenic seedlings incca1-11(orange),lhy21(green),cca1-11 lhy21(purple) and Ws (black) backgrounds, which were subjected to control (e) or cold (f) treatments. One of three replicate experiments (× 10,000 counts per second±s.e.m.,n=16 individuals per transgenic line, three independent transgenic lines were examined) is shown. Figure 3: The circadian clock regulates the rhythmic expression of ACD6 and COR78 . ( a , b ) Bioluminescent activities of pACD6(Ws):LUC in T3 transgenic seedlings that were treated with SA (red) and the control (black; a ) and of pCOR78(Ws):LUC in T3 transgenic seedlings that were treated with cold (red) and the control (black; b ). ( c , d ) Altered bioluminescent activities of pACD6(Ws):LUC in T3 transgenic seedlings in cca1-11 (orange), lhy21 (green), cca1-11 lhy21 (purple) and Ws (black) backgrounds, which were sprayed with water (control, c ) or SA ( d ). ( e , f ) Altered bioluminescent activities of pCOR78(Ws):LUC in T3 transgenic seedlings in cca1-11 (orange), lhy21 (green), cca1-11 lhy21 (purple) and Ws (black) backgrounds, which were subjected to control ( e ) or cold ( f ) treatments. One of three replicate experiments (× 10,000 counts per second±s.e.m., n =16 individuals per transgenic line, three independent transgenic lines were examined) is shown. Full size image Stress-responsive expression as a predictor for heterosis The diurnal regulation of stress-responsive genes could provide a basis for natural variation among diverse ecotypes tested ( Fig. 4a,b , Supplementary Table 3 and Supplementary Fig. 5a–d ), which is consistent with their wide-geographical distributions [12] . For example, in C24 (Coimbra, Portugal) and Cvi (Cape Verde Islands), abiotic genes were poorly expressed ( Fig. 4a,b and Supplementary Fig. 5c,d ), but biotic genes were highly expressed at ZT18, which correlated with higher SA levels and more necrotic lesions on mature leaves in C24 than in Col ( Fig. 1c ) [26] , [40] . This is because these ecotypes are adapted to warmer environments with relatively more pathogens [40] . However, in Col (Columbia, USA), L er (Germany) and Ws (Russia), where the plants are presumably adapted to colder climates, COR78 and COR47 were highly expressed at ZT9 ( Fig. 4b and Supplementary Fig. 5d ), but ACD6 and PR1 were poorly expressed [26] , [41] , [42] ( Fig. 4a and Supplementary Fig. 5c ). Interestingly, no ecotype tested showed low expression levels of both biotic and abiotic stress-responsive genes, indicating that the basal level of stress responses reflects a genetic basis for a given ecotype’s adaptation to its local environment [12] , [13] . Thus, the overall repression of stress-responsive genes of both parental origins is unique in the hybrids, which could affect heterosis. This also suggests that natural variation in stress-responsive-gene expression between parents could be used to predict the level of heterosis. 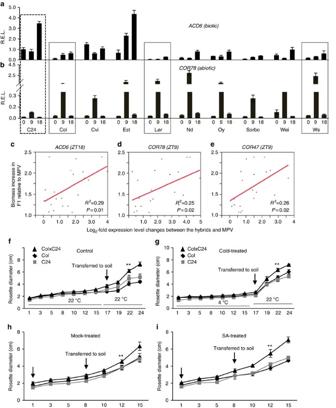Figure 4: Stress-responsive gene expression levels as predictors for heterosis and effects of cold stress and SA on growth rate. (a,b) Relative expression levels (R.E.L.) ofACD6(a) andCOR78(b) in 10 ecotypes at ZT0, ZT9 and ZT18. Values are averages from three biological replicates (±s.d.). C24 (dashed-box) has higherACD6and lowerCOR78expression levels than Col, Lerand Ws (grey boxes). (c–e) Biomass increase relative to MPV (yaxis) in various hybrids was plotted against absolute values of the log2-fold expression level changes (xaxis) in different stress genes at three time points (ZT0, 9 and 18). Scatter plots forACD6at ZT18 (c),COR78at ZT9 (d) andCOR47at ZT9 (e). Regression lines (red) were statistically significant forACD6at ZT18 (c),COR78at ZT9 (d) andCOR47at ZT9 (e). Data used to perform regression analyses were shown inSupplementary Table 3, and detailed results of the analysis were included inSupplementary Data 3. (f,g) Rosette diameters of seedlings (n=15 plants averaged per replicate) that were grown at 22oC (f) or 4oC (g) for 17 days and transferred to grow in soil for another 8 days at 22 °C. (h,i) Rosette diameters of seedlings (n=15 plants averaged per replicate) that were mock-treated (h) or treated with SA twice (indicated by arrows; SA) (i) and were transferred to soil for another 8 days. Values were averaged from three biological replicates (mean±s.d.). Single and double asterisks indicate statistically significant levels ofP<0.05 andP<0.01 using two-tailed Student’st-test (compared with MPV), respectively. Figure 4: Stress-responsive gene expression levels as predictors for heterosis and effects of cold stress and SA on growth rate. ( a , b ) Relative expression levels (R.E.L.) of ACD6 ( a ) and COR78 ( b ) in 10 ecotypes at ZT0, ZT9 and ZT18. Values are averages from three biological replicates (±s.d.). C24 (dashed-box) has higher ACD6 and lower COR78 expression levels than Col, L er and Ws (grey boxes). ( c – e ) Biomass increase relative to MPV ( y axis) in various hybrids was plotted against absolute values of the log 2 -fold expression level changes ( x axis) in different stress genes at three time points (ZT0, 9 and 18). Scatter plots for ACD6 at ZT18 ( c ), COR78 at ZT9 ( d ) and COR47 at ZT9 ( e ). Regression lines (red) were statistically significant for ACD6 at ZT18 ( c ), COR78 at ZT9 ( d ) and COR47 at ZT9 ( e ). Data used to perform regression analyses were shown in Supplementary Table 3 , and detailed results of the analysis were included in Supplementary Data 3 . ( f , g ) Rosette diameters of seedlings ( n =15 plants averaged per replicate) that were grown at 22 o C ( f ) or 4 o C ( g ) for 17 days and transferred to grow in soil for another 8 days at 22 °C. ( h , i ) Rosette diameters of seedlings ( n =15 plants averaged per replicate) that were mock-treated ( h ) or treated with SA twice (indicated by arrows; SA) ( i ) and were transferred to soil for another 8 days. Values were averaged from three biological replicates (mean±s.d.). Single and double asterisks indicate statistically significant levels of P <0.05 and P <0.01 using two-tailed Student’s t -test (compared with MPV), respectively. Full size image To test the relationship between natural variation of stress responses and heterosis in hybrids, we performed a regression analysis between the mean increase in biomass relative to the MPV as the dependent variable and the expression level difference for a given stress-responsive gene between the parents at different time points as the independent predicting variable ( Fig. 4c–e , Supplementary Table 3 and Supplementary Fig. 5e–p ). We found that expression differences of the stress-responsive genes between parental ecotypes at certain times of day, including ACD6 at ZT18, COR78 at ZT9 and COR47 at ZT9 ( Figs. 4c–e ), were significantly correlated with biomass heterosis ( P <0.05, Supplementary Data 3 ). This indicates that the timing of measurement of expression in the parents is crucial for accurately predicting the level of heterosis based on expression differences of stress-responsive genes. Using data from an independent study, we compared quantitative trait loci (QTL) for biomass heterosis [43] with the DEGs in the hybrids ( Supplementary Table 4 ). The DEGs overlapped significantly with two QTL regions using both hypergeometric and non-parametric randomization tests ( P =0.01). Moreover, many stress-responsive genes including COR15A and PR2 , both of which were downregulated in the hybrids, coincided within the QTL regions, suggesting a potential role of these candidate genes underlying the QTL of biomass heterosis. According to the hypothesis that genetic distance plays a role in heterosis, higher levels of heterosis could be obtained from the parents with larger expression differences in stress-responsive genes. For example, the hybrids between Col and C24 with larger COR78 and ACD6 expression differences ( Fig. 2 ) displayed higher heterosis ( Fig. 1a ). Using this concept, we predicted two additional high-vigour F1 hybrids (C24XL er and C24XWs; Figs. 5a–d ), which correlated with larger ACD6 and COR78 expression differences between the parents (C24 versus L er and C24 versus Ws) ( Fig. 4a,b ). In contrast, if the parents had similar levels of ACD6 and COR78 expression (for example, Col versus Ws and Col versus L er ; Supplementary Fig. 6a–d ), their F1 hybrids displayed relatively low levels of heterosis (ColXWs and ColXL er ; Fig. 5e,f and Supplementary Fig. 6e,f ), as reported elsewhere [29] , [30] , [31] . Moreover, in the high-vigour hybrids, both COR78 and ACD6 were repressed at most time points ( Supplementary Fig. 6g–j ), whereas in low-vigour hybrids, COR78 and ACD6 , were generally repressed but also upregulated at several time points ( Supplementary Fig. 6a–d ). Another F1 hybrid (EstXCol) displayed high biomass heterosis ( Supplementary Fig. 6k ), which correlated with repression of both ACD6 and COR78 ( Supplementary Fig. 6l,m ). 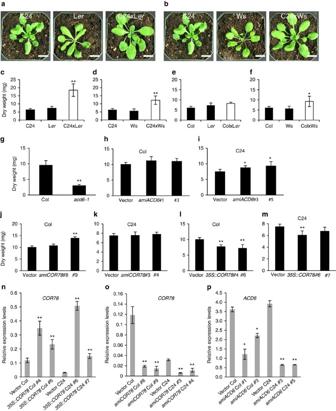Figure 5: Effects of knockdown or overexpression of abiotic and biotic genes on biomass. (a) Rosettes of 3-week-old plants in F1(C24 × Ler) and its parents C24 and Ler. (b) Rosettes of 3-week-old plants in F1(C24 × Ws) and its parents C24 and Ws. Scale bars, 1 cm for all images. (c–f) Biomass of rosettes from 3-week-old seedlings in high-vigour crosses C24XLer(c) and C24XWs (d) and low-vigour crosses ColXLer(e) and ColXWs (f). Values were averaged from three biological replicates (±s.d.). (g) Biomass of Col andacd6-1hyperactive mutant. (h,i) Dry weight (mg) of transgenicamiRACD6lines in Col (h) and in C24 (i). (j,k) Dry weight (mg) of transgenicamiRCOR78lines in Col (j) and in C24 (k). (l,m) Dry weight (mg) of transgenic35 S:COR78lines in Col (l) and in C24 (m). (n–p) Relative expression levels ofCOR78expression in overexpression lines (n) and in artificial microRNA (amiRNA) lines (o) and ofACD6in amiRNA lines (p). Values were averaged from three biological replicates (±s.d.). Single and double asterisks indicate statistical significance levels atP<0.05 andP<0.01 using two-tailed Student’st-test, respectively, compared with the transgenic control (vector). Figure 5: Effects of knockdown or overexpression of abiotic and biotic genes on biomass. ( a ) Rosettes of 3-week-old plants in F1(C24 × L er ) and its parents C24 and L er . ( b ) Rosettes of 3-week-old plants in F1(C24 × Ws) and its parents C24 and Ws. Scale bars, 1 cm for all images. ( c – f ) Biomass of rosettes from 3-week-old seedlings in high-vigour crosses C24XL er ( c ) and C24XWs ( d ) and low-vigour crosses ColXL er ( e ) and ColXWs ( f ). Values were averaged from three biological replicates (±s.d.). ( g ) Biomass of Col and acd6-1 hyperactive mutant. ( h , i ) Dry weight (mg) of transgenic amiRACD6 lines in Col ( h ) and in C24 ( i ). ( j , k ) Dry weight (mg) of transgenic amiRCOR78 lines in Col ( j ) and in C24 ( k ). ( l , m ) Dry weight (mg) of transgenic 35 S:COR78 lines in Col ( l ) and in C24 ( m ). ( n – p ) Relative expression levels of COR78 expression in overexpression lines ( n ) and in artificial microRNA (amiRNA) lines ( o ) and of ACD6 in amiRNA lines ( p ). Values were averaged from three biological replicates (±s.d.). Single and double asterisks indicate statistical significance levels at P <0.05 and P <0.01 using two-tailed Student’s t -test, respectively, compared with the transgenic control (vector). Full size image Hybrids have a timed stress-response strategy It is paradoxical that in the absence of stress, stress-responsive genes were repressed in the hybrids, and yet hybrids are generally more tolerant than parents to stresses [41] , [42] . To address this paradox, we tested growth vigour and stress responses in the hybrids and their parents during short- and long-term stress treatments. After short-term cold shock treatment at ZT0 or ZT15 (see Methods and Supplementary Fig. 7 ), both COR78 and COR15A transcripts were transiently induced in ColXC24 hybrids and their parents ( Supplementary Fig. 8a–d ). Cold treatment caused a greater increase in gene expression at ZT15 than ZT0 ( Supplementary Fig. 8 , a versus b and c versus d) because of gating of induction by the circadian clock and diurnal regulation of stress responses [19] , [21] , [22] . Interestingly, higher than MPV induction of stress-responsive genes in the hybrids occurred only at some specific time points (for example, COR15A at ZT3 and ZT9 and COR78 at ZT9). Similarly, after SA treatment, both ACD6 and PR1 were also expressed at higher levels at ZT15 than at ZT0 ( Supplementary Fig. 8e–h ). In the hybrids, induction of PR1 and ACD6 was delayed for a few hours after SA treatment, but ultimately reached a level higher than the MPV at several time points. Under long-term stress (cold or SA) conditions (see Methods and Supplementary Fig. 7 ), hybrids maintained higher relative growth rates (RGR) than their parents ( Fig. 4f–i ). After removal from stress conditions the RGR of hybrids accelerated more than that of the parents, consistent with increased protection from freezing damage during cold stress [41] , [42] . As a result, hybrids accumulated more biomass than parents ( Supplementary Fig. 8i,j ). Hybrids also showed higher than MPV induction of cold-responsive genes at certain times after 2 weeks growing in the cold, although this trend was less obvious after the long-term treatment with SA ( Supplementary Fig. 8k–n ). These data collectively suggest that stress-responsive genes, which are normally repressed in the hybrids, can be rapidly induced at certain time points under stress, which we propose may preserve energy and metabolism to promote growth in the presence of stress. This is reminiscent of the tradeoff between growth and fitness in diploids [24] , [25] , [26] . Effects of stress-responsive genes on biomass It is well established that constitutive defense responses decrease biomass, growth rate and seed production [28] , [44] , and R genes reduce fitness in the absence of pathogens [24] , [45] . To determine whether the repression of stress-responsive genes in the hybrids could promote growth vigour, we investigated the effects of repressing and overexpressing ACD6 and COR78 on biomass in Col and C24 ecotypes ( Fig. 5g–m ). The dominant-negative mutant acd6-1 accumulated less biomass than the wild type because of the production of higher amounts of SA and spontaneous cell death [26] ( Fig. 5g ). Conversely, knockdown of ACD6 ( amiACD6 ) using artificial microRNAs showed a modest but nonsignificant increase in biomass relative to Col ( Fig. 5h ), whereas amiACD6 in C24 showed significant increases in biomass ( Fig. 5i ). This is probably because the basal expression level of ACD6 is low in Col, and SA levels are naturally elevated in C24 (refs 40 , 46 ). Overexpressing COR78 in either Col or C24 caused biomass reductions at statistically significant levels ( Fig. 5l,m ), and repressing COR78 increased biomass in Col but not in C24 ( Figs. 5j,k ). This is likely because the basal expression level of COR78 is low in C24, and expression levels of cold stress-responsive genes are high in Col [41] , [42] , [47] . Thus, repressing COR78 has a smaller effect in C24 than in Col. Biomass increase or reduction in individual transgenic lines was anticorrelated with expression levels of ACD6 and COR78 , respectively ( Fig. 5n–p ). Thus, reducing or increasing expression of a single stress-responsive gene in diploids can alter biomass, and simultaneous suppression of many of these genes in hybrids could lead to biomass heterosis. Epigenetic reprogramming of hybrids The available data indicate that natural variation and circadian regulation of stress-responsive gene expression is correlated with heterosis. Different ecotypes experience diurnal and seasonal changes in their corresponding environments, leading to differences in circadian regulation of stress-responsive gene expression. We propose that over time, ‘long-term’ adaptation to the local environment results in genetic and epigenetic variations between parents, which is reprogrammed in hybrids to change the expression of circadian regulators [17] , [48] and stress-responsive genes, and possibly metabolites [42] , [49] , leading to heterosis. Consistent with the role of epigenetic variation in heterosis [18] , the overall levels of CG, CHG and CHH (H=A, T or C) methylation in many genes, including biotic and abiotic stress-responsive genes ( Fig. 6a,b ), were generally increased in hybrids compared with parents [48] ( Fig. 6c–k ). These results are reminiscent of dynamic changes in transposon methylation that can regulate the expression of neighbouring genes in response to biotic stress [50] and of changes in CHH methylation that mediate circadian gene expression and heterosis in reciprocal F1 hybrids [18] . In DNA methylation mutants, the circadian-clock genes, CCA1 and LHY, and stress-responsive genes, including ACD6 and PR1, are upregulated, indicating repression of these genes by DNA methylation [51] . Consequently, increased methylation levels in hybrids selectively repress stress-responsive genes [48] . 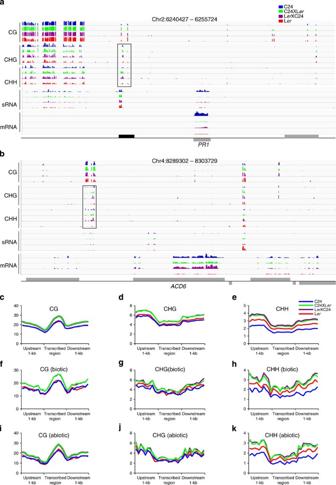Figure 6: Analysis of DNA methylation in stress-related genes. (a,b) Sequence densities and distributions of CG, CHG and CHH (H=A, T or C) methylation, small RNA and mRNA in the vicinity ofPR1(a) andACD6(b) genomic regions. Grey boxes are genes and black boxes are transposons. Changes in CHG and CHH methylation between F1 reciprocal hybrids and their parents (Lerand C24) are boxed. Genomic coordinates are shown above each diagram. (c–e) Percentage (%,yaxis) of CG (c), CHG (d) and CHH (e) methylation (H=A, T or C) levels in all genes. (f–h) Percentage (%,yaxis) of CG (f), CHG (g) and CHH (h) methylation levels in all biotic stress-responsive genes. (i–k) Percentage (%,yaxis) of CG (i), CHG (j) and CHH (k) methylation levels in all abiotic stress-responsive genes.xaxis: positions relative to the transcribed region. Data were extracted from the published paper48. Figure 6: Analysis of DNA methylation in stress-related genes. ( a , b ) Sequence densities and distributions of CG, CHG and CHH (H=A, T or C) methylation, small RNA and mRNA in the vicinity of PR1 ( a ) and ACD6 ( b ) genomic regions. Grey boxes are genes and black boxes are transposons. Changes in CHG and CHH methylation between F1 reciprocal hybrids and their parents (L er and C24) are boxed. Genomic coordinates are shown above each diagram. ( c – e ) Percentage (%, y axis) of CG ( c ), CHG ( d ) and CHH ( e ) methylation (H=A, T or C) levels in all genes. ( f – h ) Percentage (%, y axis) of CG ( f ), CHG ( g ) and CHH ( h ) methylation levels in all biotic stress-responsive genes. ( i – k ) Percentage (%, y axis) of CG ( i ), CHG ( j ) and CHH ( k ) methylation levels in all abiotic stress-responsive genes. x axis: positions relative to the transcribed region. Data were extracted from the published paper [48] . Full size image On the basis of our findings, we propose a general role for the repression of stress-responsive genes by both epigenetic mechanisms and circadian clock regulators in hybrids to promote biomass heterosis under non-stress conditions. Under stress conditions, hybrids induce expression of repressed stress-responsive genes at certain times of the day to combat the effects of stress and recover faster than their parents after stress conditions are removed. This role for the timing of stress responses in biomass heterosis is reminiscent of the connection between altered clock gene expression and growth vigour in Arabidopsis allopolyploids and diploids [17] . In particular, repressing CCA1 expression peaks in TOC1::cca1 (RNAi) transgenic plants during the day increases starch content and biomass, while overexpressing TOC1::CCA1 in the transgenic plants decreases starch content and biomass. These findings provide a direct link between circadian regulators and biomass heterosis through promoting the clock output pathways of photosynthesis and starch metabolism [10] , [17] . Our current data suggest that this clock-heterosis link involves another clock output pathway, namely, stress responses. In addition to regulation by the circadian clock, stress-responsive genes are epigenetically regulated in the hybrids. Our model of balancing stress response to promote heterosis can help to explain both heterosis and hybrid necrosis ( Fig. 7 ). Hybrid necrosis, as previously reported [52] , was likely caused by the induction of stress-responsive genes. Indeed, expression of several stress-responsive genes including PR1 , PR2 and PR5 is elevated in these necrotic hybrids [52] . However, the higher-vigour hybrids have a better-timed stress-response strategy whereby stress-responsive genes are generally repressed under non-stress conditions and selectively induced at certain times under the stress, thus balancing the tradeoff between a rapid requirement for stress responses and long-term maintenance of growth vigour. This stress-response strategy is inherited from adaptively divergent ecotypes, with more competitive species having lower levels of constitutive expression of stress-responsive genes but higher levels of inducible resistance [28] . Hybrids may simply have exploited this adaptive response. Hybrid plants recovered faster than their parents after encountering stresses, suggesting that hybrids have a higher potential to promote growth by regulating stress responses under both stress and non-stress conditions. Using a couple of stress-responsive genes in several time points, we could accurately predict the biomass heterosis on the basis of their expression levels between different pairs of parental lines. We expect that the predictability could be dramatically improved if multiple genes and many more time points are implemented in the statistical model. In conclusion, we suggest that this link between natural variation, circadian regulation of stress-responsive genes and heterosis could guide the selection of parents to improve hybrid production of plants and animals. 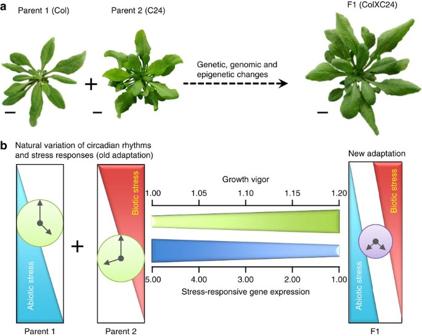Figure 7: A model for altered stress-responsive gene expression and growth vigour in hybrids. (a) An example of an F1 (ColXC24) hybrid showing growth vigour compared with the parents, Col and C24 (scale bars, 1 cm). Natural variation of circadian rhythms and stress responses is associated with the adaptation of each ecotype to local environments. (b) Parent 1 and parent 2 who have adapted to different environments require high levels of gene expression in response to abiotic (parent 1) or biotic (parent 2) stress, which is partly mediated by circadian rhythms (clock symbols). Parent 1 and parent 2 do not reach the full growth potential, probably because of the fitness cost in response to the stress in respective adaptive environments. In F1 hybrids, the expression of both biotic and abiotic stress-responsive genes is compromised, which we propose leads to increased levels of growth vigour. Figure 7: A model for altered stress-responsive gene expression and growth vigour in hybrids. ( a ) An example of an F1 (ColXC24) hybrid showing growth vigour compared with the parents, Col and C24 (scale bars, 1 cm). Natural variation of circadian rhythms and stress responses is associated with the adaptation of each ecotype to local environments. ( b ) Parent 1 and parent 2 who have adapted to different environments require high levels of gene expression in response to abiotic (parent 1) or biotic (parent 2) stress, which is partly mediated by circadian rhythms (clock symbols). Parent 1 and parent 2 do not reach the full growth potential, probably because of the fitness cost in response to the stress in respective adaptive environments. In F1 hybrids, the expression of both biotic and abiotic stress-responsive genes is compromised, which we propose leads to increased levels of growth vigour. Full size image Plant materials and growth conditions Plant materials include the following A. thaliana ecotypes, which were used to generate F1 hybrids; C24, Columbia (Col), Cvi-0 (CS22614), Est-1 (CS22629), L er , Nd-1 (CS22619), Oy-0 (CS22658), Sorbo (CS22653), Wei-0 (CS22622) and Ws. Crossing was carried out as previously described [29] . The acd6-1 hyperactive mutant was a generous gift from Dr Detlef Weigel (Max Planck Institute for Developmental Biology, Tübingen, Germany) and cca1-11 (CS9378), lhy21 (CS9379) and cca1-11lhy21 (CS9380) T-DNA insertion mutants in the Ws background were obtained from the Arabidopsis Biological Resource Center (ABRC). All plants were grown under a 16/8-h light/dark cycle with temperatures of 22 °C (light) and 20 °C (dark) on soil, and rosette leaves from ∼ 3-week-old plants before flowering were collected for RNA analysis, unless otherwise noted. For qRT–PCR validation, plants were grown in three biological replicates, and leaves were harvested every 3 h for two diurnal cycles (48 h). For plant transformation, 4- to 5-week-old plants were used for Agrobacterium tumefaciens -mediated transformation through floral dipping [53] . Biomass measurement Biomass was measured after drying rosettes before bolting at 80 °C for 24 h as previously described [29] , and the number of plants per replicate is indicated in Figure legends. Trypan blue staining Trypan blue staining was performed as described previously [54] with minor modifications. Briefly, the staining solution was prepared by adding 20 mg of Trypan blue to 40 ml of lactophenol solution for a final concentration of 0.5 mg ml −1 . Leaves were incubated for 3 h in a sufficient amount of solution to immerse the tissue. The tissue was then cleared in a sufficient amount of chloral hydrate solution to cover the tissue (25 g of chloral hydrate per 10 ml water) for 30 min. mRNA-seq library preparation Total RNA was isolated from mature leaves (3-week-old A. thaliana plants) before bolting using plant RNA purification reagent (Invitrogen). The integrity of extracted RNA was analysed by resolving 1 μg RNA in a 1%-formaldehyde denaturing agarose gel. An aliquot of 10 μg total RNA was used to prepare mRNA-seq libraries using the Illumina mRNA-seq sample preparation kit (Illumina). Libraries with a range of 200±25 bp were excised and amplified for subsequent cluster generation and massively parallel sequencing using the Illumina Genome Analyzer GII with read lengths of 85 bp. mRNA-seq read mapping and expression quantification mRNA-seq reads from 12 libraries (Col, C24, ColxC24 and C24xCol at three time points) were mapped to the TAIR9 genome and cDNA sequence using BFAST ( http://bfast.sourceforge.net ) [55] . Transcript levels were quantified by counting reads per kilobase per million mapped reads (RPKM) as previously described [32] . First, all unique reads without alternative splice isoforms were used to calculate a preliminary RPKM. Second, unique reads with isoform exons were weighted using the preliminary RPKM. Final RPKMs were calculated by combining the unique and weighted-multiple mapped reads. We used the primary isoforms for further analysis, although RPKM values for all isoforms are available (see below). These isoforms could indicate a role for splicing variants of circadian clock genes in a temperature-dependent mechanism [56] . The RNA-sequence data have been deposited at GEO ( http://www.ncbi.nlm.nih.gov/geo/ ) with the accession number GSE51578 . Bioinformatics analyses Differentially expressed genes were identified using the R-package DEGseq with a log 2 fold change >|0.5| and a FDR-corrected P value ( q value)<0.05 ( Supplementary Data 1 ) [57] . Heat maps were generated using Gene-E ( http://www.broadinstitute.org/cancer/software/GENE-E/ ), and clustering was performed using the default settings (one minus Pearson correlation). RPKM values used to generate heat maps are located in Supplementary Data 2 , along with locations of EE and CBS motifs and circadian correlations of the genes displayed in the heat maps [58] . GO analysis was performed and figures were generated using the agriGO website [59] . The hypergeometric test was used to identify enriched (FDR-adjusted P value<0.05) GO categories relative to the genome background. Genes were identified as biotic or abiotic stress-responsive using GO term analysis, followed by manual removal of uncharacterized genes to ensure that the classifications were accurate. Single-nucleotide polymorphism (SNP) data for C24 were obtained from the Arabidopsis 1001 genomes database ( http://1001genomes.org/ ). Reads mapped to regions containing SNPs were extracted and then assigned to reads from Col or C24 according to the SNP database. The total RPKM value in hybrids was split to Col and C24 alleles based on the ratio between the number of reads mapped to either Col and C24 (ref. 32 ). To calculate cis- and trans- effects, a previously published strategy was employed [32] . Log 2 -transformed ratios were used to estimate allelic expression divergence, such that gene-expression divergence (A) between ecotypes was calculated by log 2 (Col/C24) and the allelic ratio in the hybrids by log 2 (F1Col/F1C24). Genes that showed different expression between parents (log 2 fold change>|1|), but the same allelic expression within the hybrid (log 2 fold change<|0.5|), was considered to be caused by only trans -effects. A gene was considered having only cis -effects if the ratio of parental expression was equal to the allelic expression in hybrid or allotetraploid (A=B, log 2 fold change<|0.5|). Circadian-regulated genes were identified by comparing a given data set (that is, DEG or MPV gene lists in parents and hybrids, respectively) with the intersection of two different microarray experiments (Covington+Edwards intersection [39] ). Integrative Genomics Viewer (IGV) was used to display publically available mRNA-seq, sRNA-seq and methylation data from ref. 48 (GSE34658). Genes were identified as having a higher methylation level than the MPV if average methylation differences were 0.1 or greater for CG and CHG contexts and 0.05 or greater for CHH contexts, similar to the criteria used by in ref. 48 . For QTL analysis, genes present in the QTL intervals in Supplementary Table 4 from ref. 43 were tested for significant overlap with DEGs using the GeneSect Tool, which implements a non-parametric randomization test that can determine whether the overlap between two gene lists is higher or lower than expected by chance, from the Virtual Plant website [60] , as well as the hypergeometric test in R. RNA extraction and qRT–PCR Tissue collected for gene expression analysis was from plants before bolting (3-week-old plants unless noted otherwise) at indicated ZT (ZT0=dawn) [61] . Total RNA was extracted using Concert Plant RNA Reagent (Invitrogen) and digested with RQ1 RNase-Free DNase (Promega) according to the manufacturer’s instructions. cDNA was synthesized using 1 μM oligo dT (12–18) primer (GeneLink) from 1 μg DNase-treated RNA using the Omniscript RT Kit (Qiagen) according to the manufacturer’s instructions. For qRT–PCR, FastStart Universal SYBR Green Master (Rox; Roche Applied Science) was used for PCR in the presence of gene-specific primers and 2 μl of diluted cDNA template. Expression levels of target genes were normalized against transcript levels of ACT7 (At5g09810) and relative expression levels of transcripts were calculated. The primer sequences are listed in Supplementary Table 5 . Plasmid constructs For luciferase reporter constructs, genomic DNA from Col, C24 and Ws was used to amplify ACD6 and COR78 promoter regions. SNPs between Col and C24 promoter and coding regions were identified using Polymorph ( http://polymorph-clark20.weigelworld.org/index.php ). The amplified fragments were cloned into pGEM-T vector (Promega) for sequence verification. The Promoter:LUC plasmid constructs were generated by inserting the luciferase gene between the restriction enzyme sites NcoI and BamHI in the pFAMIR plasmid (from the laboratory of Dr Ramin Yadegari, University of Arizona). For 35S-driven overexpression constructs, the transcribed region of COR78 from Col or C24 was cloned into the pF35 SE vector (A vector for 35S-driven gene expression, courtesy of Dr Ramin Yadegari, University of Arizona) between RsrII and AatII restriction sites. Artificial miRNAs were designed using the WMD3 web app ( http://wmd3.weigelworld.org/cgi-bin/webapp.cgi ) against a conserved region in Col and C24 and then amplified using the pRS300 vector as a template. The amplified fragments were cloned into pGEM-T vector (Promega) for sequence verification. The artificial miRNAs were then cloned into the pF35SE vector between RsrII and AatII restriction sites for amiACD6 and between XmaI and AatII restriction sites for amiCOR78 . All constructs were individually cloned into Agrobacterium strain GV3101 for plant transformation and seeds were screened on 1% (w/v) agar with Murashige and Skoog (MS) media containing 7.5 mg l −1 phosphinothricin. The primer sequences are listed in Supplementary Table 5 . Luciferase assays Plants containing either ACD6:LUC or COR78:LUC constructs were analysed using a Packard TopCount luminometer as previously described [62] . Seeds were sterilized with bleach and 75% ethanol and plated on 1% (w/v) agar with MS media containing 7.5 mg l −1 phosphinothricin. Seeds were stratified 2 days in the dark at 4 °C and then transferred into 16-h light and 8-h dark cycles for 7 days, and then transferred to MS containing no selection for 3 days. Seedlings were transferred to white microtitre plates (Nunc, Denmark) containing agar MS medium plus 30 g sucrose/L and 30 μl of 0.5 mM luciferin (Gold Biotechnology). Microtitre plates were covered with clear plastic MicroAmp sealing film (Applied Biosystems, Foster City, CA) in which holes were placed above each well for seedling gas exchange. One day after addition of luciferin, plates were moved to the TopCount and interleaved with two clear plates to allow light diffusion to the seedlings. All luciferase data were analysed using the Biological Rhythm Analysis Software System ( www.amillar.org ). All period estimates were performed on rhythms from 24 to 120 h using fast Fourier transform–nonlinear least squares (FFT–NLLS) analysis [63] . Regression analysis Regression analysis was performed using JMP 10 (JMP, Version 10, SAS Institute Inc., Cary, NC, 1989–2007) with the default parameters and all graphs were generated using JMP. Data used for the regression analysis are in Supplementary Table 3 , and detailed results can be found in Supplementary Data 3 . Cold- and SA-treatment experiments The scheme for stress experiments is shown in Supplementary Fig. 7 . For cold induction of gene expression (cold shock), six 2-week-old seedlings (three seedlings were used per replicate) were removed from agar media and were placed into 5 ml culture tubes containing room-temperature liquid MS media with 3% sucrose 24 h before cold treatment [37] . Cold treatment was performed by placing the tubes in ice or leaving at 22 °C for the control. After 60 min, tubes containing seedlings were placed back into 22 °C and then whole seedlings (excluding roots) were snap-frozen in liquid nitrogen at the ZT times listed in Supplementary Fig. 7 . For SA induction of gene expression, 2-week-old seedlings growing on agar media were sprayed with 1 mM SA (Sigma-Aldrich). After 60 min, whole seedlings (excluding roots) were snap-frozen in liquid nitrogen for the first time point, and then at the subsequent ZT times listed in Supplementary Fig. 7 . For longer-term cold-stress application, 2-week-old seedlings growing on agar media were placed into a 4 °C growth chamber of the same light intensity as control seedlings that were left at 22 °C. Every 2–3 days, seedlings were photographed and rosette diameter was quantified using ImageJ [64] .Every 2–3 days, seedlings were photographed and rosette diameter was quantified using ImageJ [64] . After 2 weeks, seedlings were snap-frozen in liquid nitrogen at ZT0, ZT9 and ZT15. A batch of seedlings was transferred to soil, placed at 22 °C to allow for recovery and rosette diameter was measured every 2–3 days. After 1 week biomass was measured. For longer-term SA treatment, 2-week-old seedlings growing on agar media were sprayed with 1 mM SA or water (control). Rosette diameter was measured every 2–3 days as described above. After 1 week seedlings were transferred to soil, sprayed with 1 mM SA again and rosette diameter was measured every 2–3 days. After one more week, seedlings were snap-frozen in liquid nitrogen at ZT0, ZT9 and ZT15 and biomass was measured. To calculate relative expression ratios, expression levels of target genes were first normalized against transcript levels of ACT7 and then the induced value was divided by the control value (indicated by a dashed line in the figures). Data of absolute values are available but not shown owing to space limitations. RGR was calculated according to RGR=(lnD 2 −lnD 1 )/ t 2 − t 1 , where D 1 and D 2 are rosette diameters at time points t 1 and t 2 , respectively [44] . How to cite this article: Miller, M. et al. Natural variation in timing of stress-responsive gene expression predicts heterosis in intraspecific hybrids of Arabidopsis . Nat. Commun. 6:7453 doi: 10.1038/ncomms8453 (2015).